Using 20-million-year-old amber to test the super-Arrhenius behaviour of glass-forming systems Fossil amber offers the opportunity to investigate the dynamics of glass-forming materials far below the nominal glass transition temperature. This is important in the context of classical theory, as well as some new theories that challenge the idea of an ‘ideal’ glass transition. Here we report results from calorimetric and stress relaxation experiments using a 20-million-year-old Dominican amber. By performing the stress relaxation experiments in a step-wise fashion, we measured the relaxation time at each temperature and, above the fictive temperature of this 20-million-year-old glass, this is an upper bound to the equilibrium relaxation time. The results deviate dramatically from the expectation of classical theory and are consistent with some modern ideas, in which the diverging timescale signature of complex fluids disappears below the glass transition temperature. P.W. Anderson said in 1995 ‘The deepest and most interesting unsolved problem in solid state theory is probably the theory of the nature of glass and the glass transition. [1] ’ This remains to be true and in the present work, we use measurements of the calorimetric and dynamic properties of an extremely stable fossil amber glass to provide new insights into the fundamentals of the nature of glass-forming materials. Vogel–Fulcher–Tammann (VFT) [2] , [3] , [4] behaviour is a classic signature of glass-forming or complex systems, and describes their equilibrium dynamics as following a super-Arrhenius behaviour that diverges at a finite temperature [5] , [6] . However, classic models [7] , [8] and some modern models [9] that predict such VFT-like behaviour have been challenged by new evidence from both theoretical [10] , [11] , [12] , [13] , [14] and experimental [15] , [16] , [17] , [18] , [19] , [20] , [21] , [22] works, which contradict such a finite temperature divergence. The difficulty of directly addressing the VFT behaviour experimentally arises owing to the ‘geological’ ages [23] required to attain equilibrium far below the glass transition temperature T g . Prior direct [15] , [16] , [17] , [18] interrogation of the equilibrium dynamics was limited to <16 °C below the T g . The VFT function describes the temperature dependence of material viscosity η or relaxation time τ : where η 0 , τ 0 , B and T ∞ are material-dependent constants. T ∞ defines the divergent point for the viscosity or relaxation time and is often related to the Kauzmann temperature [24] , which is thought to be related to the ‘ideal’ glass temperature [25] . Determining the equilibrium behaviour of a glass-forming system far below the conventional glass transition temperature has been a problem that dates at least since the time of Kauzmann [24] owing to the fact that the relaxation times grow extremely rapidly as the temperature is lowered—the previously referred to ‘geologic’ age problem [23] . While there has been some work to try to investigate the thermodynamics via extrapolation methods [26] , the dynamics remain elusive. The traditional method of addressing the sub- T g dynamics is to quench a sample from above T g to the temperature of interest and age it isothermally until it reaches equilibrium. [15] , [16] , [17] , [18] Then the equilibrium relaxation time can be determined as a function of temperature. However, this kind of measurement cannot obtain data far below T g owing to the (apparently) super-Arrhenius increase in times for the non-equilibrium glass to age into equilibrium, for example, 12 days for the mechanical response 8 K below the T g [16] . In the present work, an extremely stable (20 million year) Dominican fossil amber [27] is used to establish upper bounds on the equilibrium dynamics of a glass-forming material at temperatures to 43.6 °C below the conventional T g —sufficient to discriminate between the VFT function and the upper bounds to the equilibrium dynamics and even among non-diverging models [10] , [11] , [12] , [13] . The findings that these upper bounds deviate strongly from the ‘classical’ Vogel–Fulcher behaviour challenge classic theories [2] , [3] , [4] , [7] , [8] , some modern theories [9] and are consistent with the non-diverging models [10] , [11] , [12] , [13] . Amber sample In this work, a 20 million year (Ma) old fossil resin [27] from the Dominican Republic ( Fig. 1a ) was used to study the diverging (or not) dynamics, and the torsion rectangular mode was used to determine the stress relaxation response using a rheometer. 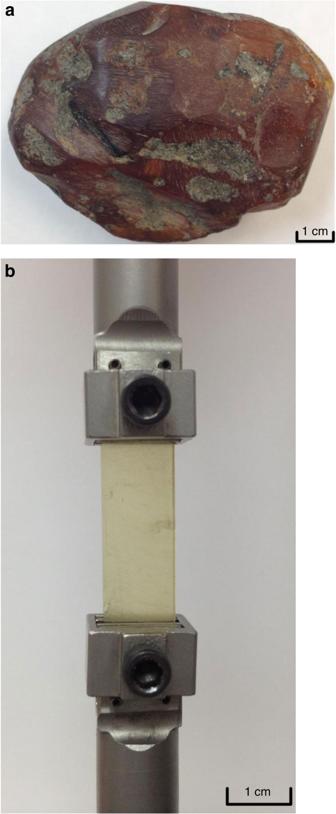Figure 1: Images of old amber. (a) As-received Dominican amber before machining. (b) Rectangular amber sample in rheometer fixtures. Figure 1b shows an amber sample in the testing fixtures. Figure 1: Images of old amber. ( a ) As-received Dominican amber before machining. ( b ) Rectangular amber sample in rheometer fixtures. Full size image The advantage of this Miocene amber compared with a normal glass-forming substance is that it has a very long-aging history at ambient conditions. This long-aging history, regardless of the full details, leads to a highly densified material [28] , which can be used to test the diverging (or not) dynamics described above. Hydrostatic weighing was used here to measure the density difference at room temperature for the 20-Ma-old amber and the same amber after thermal rejuvenation by heating to above T g followed by cooling to room temperature at 10 K min −1 . The 20-Ma-old amber has 2.1% higher density than the latter. 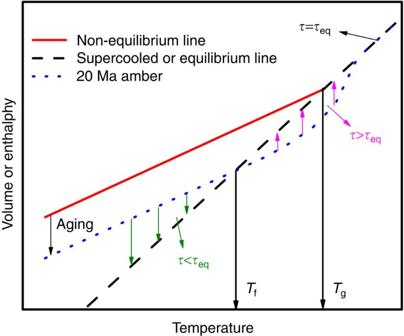Figure 2: Schematic of temperature-dependent volume or enthalphy change of glasses and supercooled liquids. This shows how extremely dense amber glass provides opportunities to obtain bounds on the equilibirium dynamics below the conventional glass transition temperature by comparing ambe sample with other glasses in a non-equilibrium state and supercooled liquids.τis the measured relaxation time andτeqis the relaxation time in equilibrium state. After 20 Ma aging, the amber has a very low fictive temperature, as depicted. Figure 2 shows a schematic of the amber volume or enthalpy beginning with ambient temperature. Importantly, even after 20 Ma, the material has not aged into equilibrium. However, as shown in the figure, as temperature is increased the volume (or enthalpy H) increases and eventually intersects with the equilibrium liquid-state extrapolated parameter. At temperatures below this intersection ( H > H eq ), the relaxation times measured should be shorter than the equilibrium times owing to the excess of volume or enthalpy relative to the equilibrium state [29] . Once the equilibrium line is crossed, as temperature increases further, the glass is in a state of lower volume or enthalpy than the equilibrium value ( H < H eq ). As a result, the relaxation times for these points should be longer than the equilibrium values of relaxation time owing to the high density [29] —hence they are upper bounds to the equilibrium value. Figure 2: Schematic of temperature-dependent volume or enthalphy change of glasses and supercooled liquids. This shows how extremely dense amber glass provides opportunities to obtain bounds on the equilibirium dynamics below the conventional glass transition temperature by comparing ambe sample with other glasses in a non-equilibrium state and supercooled liquids. τ is the measured relaxation time and τ eq is the relaxation time in equilibrium state. After 20 Ma aging, the amber has a very low fictive temperature, as depicted. Full size image DSC results In order to determine the actual calorimetric state of the amber, we performed differential scanning calorimetry (DSC) measurements. Three thermal loops were performed from −75 °C to 175 °C with the same heating/cooling rate of 10 K min −1 . It is well known that the amber resin includes both volatile and non-volatile fractions. [30] Most of the volatiles disappear during the aging process and the non-volatile parts (for example, acetogenins, fat and communic acid) become amber by free radical polymerization. Thermal analysis of different ambers, including Dominican amber, reported in the literature [31] indicates no mass loss at temperatures well above the maximum temperature of 175 ° C examined in the present investigation. The overlap of the second heating scan and the third one indicates that no physical or chemical change occurs in our heating scans to 175 °C ( Fig. 3a ). Owing to the non-isothermal sub- T g -aging history (but at temperatures more than 100 °C below the T g ) during millions of years for the amber sample, a broad endothermic shoulder [32] is observed in the first heating curve indicative of low-temperature aging and the appearance of sub- T g peaks that have not yet fully migrated to the vicinity of T g . This is somewhat different than the sharp peaks seen when aging closer to the glass transition temperature and/or when the sample has aged completely into equilibrium. 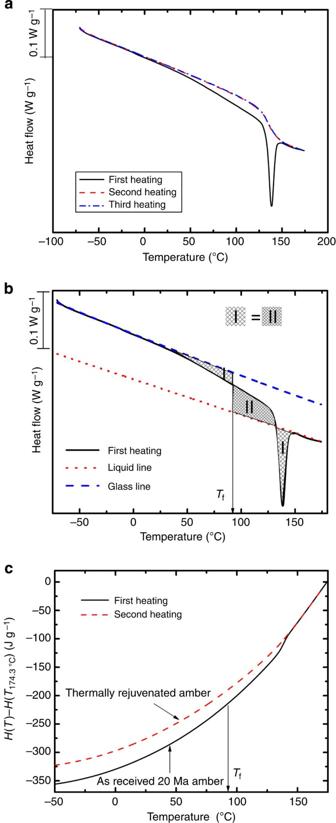Figure 3: Thermal property measurement of amber. (a) Three heating curves from DSC measurement. (b) First heating curve of amber from DSC measurement showing large enthalpy overshoot and application of Moynihan’s area matching method to obtain the amber fictive temperatureTf. (c) Relative enthalpy versus temperature curve obtained by integrating the first and second heating curves. [33] , [34] Figure 3b shows the first heating curve of the amber sample, and the fictive temperature T f for the geologically aged amber was found to be 92.6 °C using Moynihan’s method [35] such that sum of areas I equals area II (area matching method). Figure 3: Thermal property measurement of amber. ( a ) Three heating curves from DSC measurement. ( b ) First heating curve of amber from DSC measurement showing large enthalpy overshoot and application of Moynihan’s area matching method to obtain the amber fictive temperature T f . ( c ) Relative enthalpy versus temperature curve obtained by integrating the first and second heating curves. Full size image The glass transition temperature for the unaged amber on cooling at 10 K min −1 was determined to be 136.2 °C from the second heating curve by calculating the limiting fictive temperature [36] , also using Moynihan’s method [35] . By integrating the heat flow curves, we obtained the relative enthalpy versus temperature curves shown in Fig. 3c for both geologically aged and unaged amber. The first heating curve represents the properties of the amber after 20 Ma of aging, and the second one shows the amber after thermal rejuvenation. Mechanical results The 20 Ma amber was tested at different temperatures, and at each temperature, Struik’s protocol [37] was followed. As a result, we observe an interesting set of behaviours near to the T f of 92.6 °C and these confirm our hypothesis that we can obtain upper-bound relaxation times for the behaviour between T g and T f . In Fig. 4a , we compare the stress relaxation responses after 0.5 and 8 h of aging for the amber at 90 °C. Weak, but normal, physical aging behaviour is observed owing to the excess enthalpy ( T < T f ) relative to that of the equilibrium state, that is, the curve at 8 h is shifted to slightly longer relaxation times than is the curve at 0.5 h, hence the material is aging towards a lower enthalpy equilibrium state. At an aging temperature of 95 °C, however, no aging was observed during the 8 h aging ( Fig. 4b ) indicating that the amber is relatively stable at this temperature. 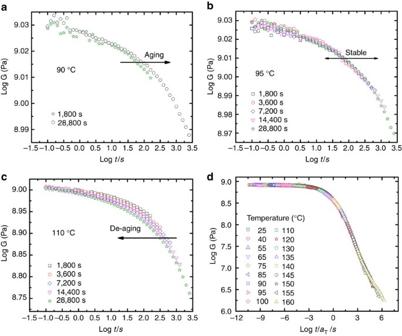Figure 4: Stress relaxation behaviour of amber at different temperatures. (a) Comparison of half-hour and 8-h stress relaxation responses at 90 °C showing normal aging behaviour. (b) Responses during 8 h measurement for amber at 95 °C and the amber is almost stable. (c) Comparison of responses at 110 °C showing shortening of relaxation times during ‘de-aging’ of sample, that is, curves provide an upper bound to equilibrium relaxation response. (d) Master curve obtained by shifting the stress relaxation curves at different temperatures onto the reference curve at 135 °C. Time–temperature superposition was applied here and shift factors (scaled relaxation times) at different temperatures obtained. Figure 4c shows the aging responses of the amber at 110 °C and we observe a ‘de-aging’ behaviour. This implies that the amber glass at 110 °C (which is well above the fictive temperature) is evolving towards the higher enthalpy state (see Fig. 2 ) and the relaxation times measured are longer than the equilibrium values and, therefore, are upper bounds to these values. Figure 4d shows the stress relaxation responses (8 h responses for temperatures below T g and 0.5 h responses for those above T g ) of amber at the different temperatures investigated. A master (or reduced) curve was obtained from time–temperature superposition [6] , [38] using the curve at 135 °C as the reference. The shift factors so-obtained are the scaled relaxation times and these are shown in Fig. 5 as a function of temperature. Figure 4: Stress relaxation behaviour of amber at different temperatures. ( a ) Comparison of half-hour and 8-h stress relaxation responses at 90 °C showing normal aging behaviour. ( b ) Responses during 8 h measurement for amber at 95 °C and the amber is almost stable. ( c ) Comparison of responses at 110 °C showing shortening of relaxation times during ‘de-aging’ of sample, that is, curves provide an upper bound to equilibrium relaxation response. ( d ) Master curve obtained by shifting the stress relaxation curves at different temperatures onto the reference curve at 135 °C. Time–temperature superposition was applied here and shift factors (scaled relaxation times) at different temperatures obtained. 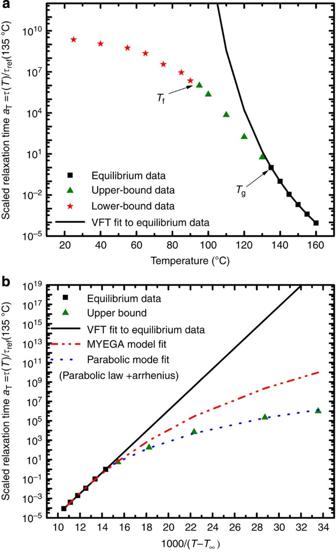Figure 5: Temperature dependence of shift factors (scaled relaxation time) comparing data and different models. (a) Scaled relaxation time versus temperature for all data, from ambient to 160 °C compared with the VFT curve fit to equilibrium data only. Data betweenTfandTgare upper bound to equilibrium response and data forT<Tfare a lower bound to the equilibrium response. (b) VFT plot of scaled relaxation time data for the temperature range fromTfto 160 °C. Full size image Figure 5: Temperature dependence of shift factors (scaled relaxation time) comparing data and different models. ( a ) Scaled relaxation time versus temperature for all data, from ambient to 160 °C compared with the VFT curve fit to equilibrium data only. Data between T f and T g are upper bound to equilibrium response and data for T < T f are a lower bound to the equilibrium response. ( b ) VFT plot of scaled relaxation time data for the temperature range from T f to 160 °C. Full size image It is now of interest to compare the results with the different possibilities of diverging and non-diverging timescales for the dynamics as one reduces the temperature below the T g and considers the upper bounds to the equilibrium relaxation time. First, the data above T g (and consequently in equilibrium) was fit to the VFT equation (equation 1). This fit and all of the data are shown in Fig. 5a . The relevant VFT parameters are: B =1071 K and T ∞ = 338.35 K. We see two things in this figure: below the T g , the extrapolation of the VFT function deviates greatly from the data—both the upper-bound data and the lower-bound data that are indicated in the plot. We emphasize that while the data within the temperature range between T f and T g is not in equilibrium, it provides an upper bound to the equilibrium relaxation time, that is, the equilibrium relaxation time is smaller or equal to our experimental data. Hence, our result actually provides powerful evidence of non-divergence of the dynamics of the amber in this temperature range. To further examine the problem, we consider two recent models in the literature that suggest that there is no finite temperature divergence of timescales below T g . We look at the predictions of the Mauro–Yue–Ellison–Gupta–Allan [11] model and the parabolic model of Chandler and co-workers [12] , [13] . Figure 5b shows a comparison between the models and the experimental data over the range of interest, that is, only the equilibrium data and the upper bound to equilibrium data. As the data are compared on a VFT plot, a straight line would describe the observed behaviour if the material continued on the VFT super-Arrhenius, finite temperature divergent path. According to the Mauro–Yue–Ellison–Gupta–Allan model [11] : Where A, C and K are fitting parameters. Although the Mauro–Yue–Ellison–Gupta–Allan model does not fit the experimental data, it shows better agreement than does the VFT model, that is, it deviates from the VFT extrapolation, though not as much as do the data. We now turn to the parabolic law model of Chandler and co-workers [12] , [13] . In this model, the relaxation times as a function of temperature are written as where J, T 0 and D are fitting parameters. T x is a crossover temperature (from low T to high T ) at which the temperature dependence of relaxation time changes from Arrhenius behaviour to super-Arrhenius response. We fit equation 3 and an Arrhenius function to the experimental data over different temperature ranges and found T x by comparing the fitting parameters, s.d. and residuals. From our data analysis, we found T x to be 135 °C, which is close to the glass transition temperature of the thermally rejuvenated amber. The activation energy below T x is 435.8 kJ mol −1 . This apparent activation energy, it does need to be remarked, is that of (essentially) a constant fictive temperature glass and represents the upper-bound relaxation times for this constant fictive temperature glass. The model itself should apply to the equilibrium system. Regardless, within these limitations, we see from the results shown in Fig. 5b that the parabolic law is in good agreement with the data, hence suggesting that T x itself may be related to the glass transition temperature measured in ordinary experiments. We note that the VFT-determined dynamic fragility [39] would be =90. We have presented the first measurements of relaxation times on an extremely stable fossil resin (20-Ma-old Miocene amber) to establish upper bounds to the temperature dependence of the dynamics of a glass-forming system far below the conventional glass transition temperature. The 20 Ma age produces an amber with 2.1% higher density than the thermally rejuvenated material and this material was found to have a calorimetric fictive temperature 43.6 °C below the T g of the thermally rejuvenated material. Hence, the upper-bound relaxation times could be probed this far into the glassy state. We suggest that there may be other ways to probe the sub- T g equilibrium dynamics (or their bounds) of glass-forming materials than through the use of extremely aged amber. One such possibility may be found in the highly stable glasses of Swallen et al . [40] They create the densified glasses by physical vapour deposition and their glasses are as much as 1.7% denser than the thermally rejuvenated glass, hence not as densified as was the 20-Ma-old amber. The Swallen et al . [40] group have reported a glass former with the fictive temperature of 31 ° C below T g , versus 43.6 ° C in the present work. However, optimization of that procedure could conceivably lead to denser materials. It may also be possible to choose a material with a very low activation energy for the equilibrium relaxation times. For example, Boehm, Ingram and Angell [34] reported an Ag 7 I 4 AsO 4 glass to have an activation energy of 210 kJ mol −1 and a T g of 63 °C, and which was aged to equilibrium within 1 year at ambient conditions (40 ° C below T g ). Even in this case, however, the next 10 °C increment requires several years and achieving equilibrium 60 °C below T g requires millennia. Finally, the experimental data for the upper-bound relaxation times of the amber over the range from T g −43.6 °C to T g provides a wide enough temperature range to evaluate the validity of different theories and leads to the conclusion that super-Arrhenius behaviour does not exist in the equilibrium state below T g for amber glass. Whether this is a universal feature of glasses requires further investigation as just suggested. We also find that the parabolic law model, including an activation energy component, from Chandler and co-workers [12] , [13] seems to provide the best description of the data of the models examined and the results suggest that the T x parameter of the model is related to the conventional glass transition temperature of the thermally rejuvenated glass. DSC measurements A Q20 calorimeter from TA Instruments was chosen to perform the DSC measurements with the same heating/cooling rate of 10 K min −1 . The scans were performed in a nitrogen atmosphere. Three thermal loops were performed from −75 °C to 175 °C. The fictive temperature T f for the geologically aged amber was obtained from the first heat curve using Moynihan’s method [35] : where C pl and C pg are the liquid and glass heat capacities, respectively. C p here is the measured value of the as-received amber heat capacity and T * is a temperature much above the transition range. The liquid and glass lines of heat capacity come from the second heating curve. Mechanical measurements The amber was cut into a rectangular shape with dimensions of 35.8 × 10.4 × 2.8 mm 3 with a band saw blade and sanded to smooth the surface. The dynamics were measured in stress relaxation tests with an ARES rheometer (TA Instruments) over a strain range from 0.03 to 3% depending on the temperature, but always in the linear regime. The geologically aged amber sample was tested from room temperature to 160 °C in a step-wise fashion (10 °C per step at temperature below T g and 5 °C per step at above T g ) in a N 2 atmosphere, and at each step in temperature, short-time stress relaxation experiments were performed following Struik’s protocol [37] after aging for successively longer times from 30 min to 8 h. In this way, we monitored the relaxation times of the glass relative to the expected bounds described above. Struik’s protocol For the non-equilibrium glassy system, Struik [37] developed a protocol to test the physical aging behaviour after a change in temperature, and we follow this protocol in our mechanical testing during our temperature-step experiments. The protocol is shown schematically in Fig. 6 . According to Struik’s protocol [37] , the testing time t d is 10% of the aging time t e so that the aging process itself will not affect the mechanical response measured, that is, a true representation of the relaxation response is obtained. Also, the aging time sequence is such that, t e,i+1 =2 t e,i , that is, a doubling with each subsequent test in order to minimize interactions between successive tests. 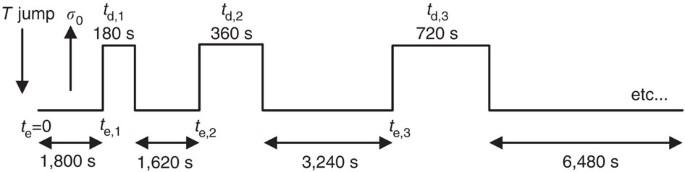Figure 6 Schematic of the Struik protocol.16 Figure 6 Schematic of the Struik protocol. [16] Full size image Time–temperature superposition Time-temperature superposition is a reduced time concept which assumes the shape of the viscoelastic response of the material under investigation, here our glass forming system, does not change with temperature. [6] , [38] . In other words, all the responses at different temperatures can be shifted to a master curve when one of them is chosen as reference. The horizontal shift factor a T is scaled relaxation time. How to cite this article: Zhao, J. et al . Using 20-million-year-old amber to test the super-Arrhenius behaviour of glass-forming systems. Nat. Commun. 4:1783 doi: 10.1038/ncomms2809 (2013).